Imperfect interface of Beclin1 coiled-coil domain regulates homodimer and heterodimer formation with Atg14L and UVRAG Beclin 1 is a core component of the Class III Phosphatidylinositol 3-Kinase VPS34 complex. The coiled coil domain of Beclin 1 serves as an interaction platform for assembly of distinct Atg14L- and UVRAG-containing complexes to modulate VPS34 activity. Here we report the crystal structure of the coiled coil domain that forms an antiparallel dimer and is rendered metastable by a series of 'imperfect' a - d' pairings at its coiled coil interface. Atg14L and UVRAG promote the transition of metastable homodimeric Beclin 1 to heterodimeric Beclin1-Atg14L/UVRAG assembly. Beclin 1 mutants with their 'imperfect' a - d' pairings modified to enhance self-interaction, show distinctively altered interactions with Atg14L or UVRAG. These results suggest that specific utilization of the dimer interface and modulation of the homodimer–heterodimer transition by Beclin 1-interacting partners may underlie the molecular mechanism that controls the formation of various Beclin1–VPS34 subcomplexes to exert their effect on an array of VPS34-related activities, including autophagy. Macroautophagy (or simply autophagy) is a cellular 'self-eating' process to remove or recycle cytosolic proteins or organelles through lysosomal degradation. The process involves the formation of double-membraned vacuoles termed autophagosomes that engulf proteins and organelles to be recycled [1] . In addition to serving as a catabolic process for recycling essential metabolic fuel under conditions of nutrient-deprived cellular stress [2] , autophagy is also involved in an array of biological and pathophysiological conditions including cancer tumorigenesis, host-pathogen immunity, embryonic development and neurodegenerative diseases [3] , [4] , [5] . Beclin 1 is the mammalian orthologue of yeast autophagy gene Atg6 (ref. 6 ), and it is the first identified mammalian autophagy gene. Previous studies found Beclin 1 to be a haploinsufficient tumour suppressor in mice, with the human Beclin 1 gene frequently deleted in breast, ovarian and prostate cancer [7] , [8] , [9] . Although the exact mechanism for Beclin 1 as a tumour suppressor remains elusive, the function of Beclin 1 in macroautophagy seems to be associated with VPS34 (vacuolar protein sorting-associated protein 34), the Class III phosphatidylinositol 3–kinase. VPS34 is the only mammalian lipid kinase that specifically phosphorylates phosphatidylinositol (PIs) at the 3 position of the inositol ring and converts them to phosphatidylinositols 3–phosphates (PI3Ps) [10] , [11] . Autophagosomes, as well as some endosomal vesicles, are particularly enriched in PI3P membrane lipids [12] . Beclin 1 tightly associates with VPS34 and directs the core Beclin 1–VPS34 assembly to a variety of cellular processes such as autophagy, endosomal trafficking and cytokinesis [13] , [14] , [15] . Emerging evidence reveals that the core Beclin 1–VPS34 complex exists in multiple forms by including different Beclin 1–interacting proteins [15] , [16] . Atg14L and UVRAG, two major activators of VPS34 activity, form stable and mutually exclusive subcomplexes with the core Beclin 1–VPS34 unit [17] , [18] , [19] , [20] . The Atg14L-containing complex is primarily involved in early stage autophagosome formation by promoting autophagosome nucleation and expansion [18] , [19] , [20] . The UVRAG-containing complex may have broader cellular functions, involved in early stage autophagy as well as late stage autophagosome maturation and fusion with the lysosome [21] . It also participates in VPS34-related endocytic trafficking and cytokinesis [22] . Beclin 1 contains three distinct functional domains, the N-terminal Bcl-2 homology 3 (BH3)-only domain, the central coiled coil (CC) domain and the carboxy-terminal evolutionarily conserved domain ECD ( Supplementary Fig. S1 ). The N-terminal BH3-only domain is involved in interaction with Bcl-family proteins to inhibit autophagy [23] , [24] , [25] . The evolutionarily conserved domain was shown to be peripherally associated with the ER and mitochondrial membrane and is essential for interaction with the VPS34 complex [26] . The CC domain of Beclin 1 is responsible for its self association in vivo [18] , [19] , [20] and for acting as a central interaction platform to engage extra factors including Atg14L, UVRAG, Bif, and Rubicon to modulate VPS34 activity [15] , [16] . However, the detailed mechanism of such interactions, particularly, how they modulate Beclin 1–VPS34 activity, is unclear. Here we present the crystal structure of the Beclin 1 CC domain and structure-based analysis of the potential mechanism through which the Beclin 1 CC domain regulates its interaction with Atg14L or UVRAG. Our data uncovers an unexpected feature of the Beclin 1 CC domain's dimer interface and suggests its role in modulating formation of multiple distinct Beclin 1–VPS34 complexes that have essential roles in controlling various membrane trafficking pathways. The 'imperfect' dimer interface of Beclin 1 CC domain The CC domain of Beclin 1 shares ∼ 25% sequence similarity with myosin-like proteins, showing a leucine-rich heptad-repeat motif as detonated by 'abcdefg' ( Fig. 1a ) [27] . This sequence feature usually induces an oligomeric CC structure, where nonpolar residues at positions a and d form the hydrophobic interface between pairs of helices. The structure of the Beclin 1 CC domain (residue 174–266) was determined by MIRAS using I and Au as two heavy-metal derivatives ( Supplementary Table S1 and Supplementary Fig. S2 ). The Beclin 1 CC domain forms a non-crystallographic dimer as a long antiparallel left-handed CC, with each peptide chain consisting of 13 heptad repeats ( Fig. 1b ). The first heptad repeat (residues 175–181) of one peptide chain packs against the 13th heptad repeat of the other peptide chain (residues 259–265). Under this arrangement, the dimeric Beclin 1 CC domain structure has an internal two-fold symmetry at the seventh heptad repeat (residue 217-223), where residues 217 and 224 on the two helices are packed against each other. The overall geometry of the Beclin 1 CC domain structure conforms to that of the classic CC ( Supplementary Fig S3 ). The full length of the CC domain is ∼ 129 Å, which roughly comprises one helical pitch made up of the two symmetry-related halves ( Fig. 1b ). 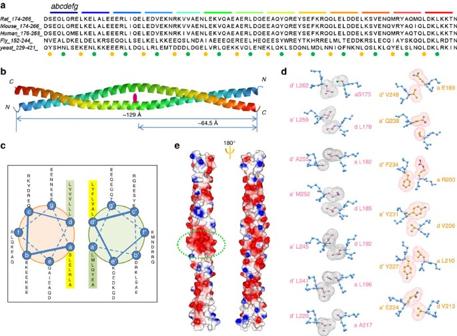Figure 1: Structure of the Beclin 1 CC Domain and its imperfect dimer interface. (a) Alignment of the Beclin 1 CC domain sequences from various species. The coloured segments and the italicabcdefgon top of the sequence indicate the heptad repeats typical of CC structure. The coloured spheres below the sequence indicate the residues ata(orange) andd(blue) position of each heptad repeat. (b) The antiparallel dimeric CC structure of the Beclin 1 CC domain. Each monomer helix is coloured in gradient varying from blue at N-terminal to red at C-terminal. The italic lettersNandCindicate the N- and C-terminal ends. The dot in the centre marks the two-fold symmetry in the CC domain structure. (c) Helical wheel presentation of the 13 heptad repeats in Beclin 1 CC domain. Only 7 heptad repeats are mapped, representing the unique half of the antiparallel symmetric dimer. (d) Close-up view of the canonical and imperfecta-d'pairings. Each residue is illustrated in ball-and-stick model. Main-chain atoms are coloured blue and side-chain atoms are coloured pink for canonical pairings or golden for imperfect pairings. Thea-d'packing is illustrated by van der Waals spheres depicting the side-chain atoms. (e) The distribution of electrostatic charges on Beclin 1 CC domain surface. Colouring scheme is according to GRASP41. The oval circle highlights the E224a-D221e'repulsive pair. Figure 1: Structure of the Beclin 1 CC Domain and its imperfect dimer interface. ( a ) Alignment of the Beclin 1 CC domain sequences from various species. The coloured segments and the italic abcdefg on top of the sequence indicate the heptad repeats typical of CC structure. The coloured spheres below the sequence indicate the residues at a (orange) and d (blue) position of each heptad repeat. ( b ) The antiparallel dimeric CC structure of the Beclin 1 CC domain. Each monomer helix is coloured in gradient varying from blue at N-terminal to red at C-terminal. The italic letters N and C indicate the N- and C-terminal ends. The dot in the centre marks the two-fold symmetry in the CC domain structure. ( c ) Helical wheel presentation of the 13 heptad repeats in Beclin 1 CC domain. Only 7 heptad repeats are mapped, representing the unique half of the antiparallel symmetric dimer. ( d ) Close-up view of the canonical and imperfect a - d' pairings. Each residue is illustrated in ball-and-stick model. Main-chain atoms are coloured blue and side-chain atoms are coloured pink for canonical pairings or golden for imperfect pairings. The a - d' packing is illustrated by van der Waals spheres depicting the side-chain atoms. ( e ) The distribution of electrostatic charges on Beclin 1 CC domain surface. Colouring scheme is according to GRASP [41] . The oval circle highlights the E224 a -D221 e' repulsive pair. Full size image Coiled coils are generally packed together in a well-defined fashion. For parallel CCs, residues at positions a and d of the heptad repeat form a-a'′ and d-d'′ packing at the dimer interface to stabilize the CC structure. For antiparallel CCs, the residue at position a on one peptide chain is packed against the corresponding residue at position d' on the other peptide to form a-d' packing. Residues at positions a and d are most frequently hydrophobic residues to pack the coils tightly together. Bulky side chains such as Tyr and Phe, or large polar side chains such as Asn or Gln are less commonly found at a or d positions. Charged residues such as Asp or Arg are extremely rare [28] . Scanning through the structure of the Beclin 1 CC domain, we noticed that the antiparallel dimeric CC structure follows the general principle described above ( Fig. 1c ). Yet, the a-d' packing at the dimer interface is far from ideal. Among the 13 unique a-d' pairs, 7 can be grouped into the category of 'canonical' pairings because they contain hydrophobic residues that form strong van del Waals interactions at the interface to stabilize the dimer ( Fig. 1d ). In particular, there are three Leu pairs (L178-L259, L192-L245, L196-L241), a signature feature of CC dimer interface that is commonly termed 'leucine zippers' for its effect to 'zip' together and stabilize the dimer structure. The remaining 6 a-d' pairs are 'imperfect' ( Fig. 1d ). Among this group, there are three a-d' pairings that contain charged residues at the a position (E189-V248, R203-F234, E224-V213). Such pairings significantly weaken dimer stability because of their unfavourable van del Waals interactions. Three extra 'imperfect' a-d' pairs contain bulky polar side chains such as Tyr (Y227 and Y231) and Gln (Q238), which also lead to weakened hydrophobic packing as compared with canonical pairs. All residues at a and d' positions are highly conserved among Beclin 1 sequences from different organisms, regardless of whether they are engaged in canonical or imperfect pairing ( Fig. 1a ). Another prominent feature of the Beclin 1 CC structure is the unusually high composition of charged amino acid residues, as reflected by its surface electrostatic potential ( Fig. 1e ). There are 26 negatively charged Asp and Glu residues, together with 16 positively charged Arg and Lys residues in the 92-residue CC domain, constituting about 50% of the total sequence. To neutralize the potentially strong Coulombic repulsion between these charged residues, there are extensive intra-chain favourable electrostatic interactions to stabilize the helical structure. We found clusters of charged triads consisting of Glu-Arg-Glu spaced at n , n +3 and n +7 positions on the helix; or clusters consisting of Glu-Asp/Glu-Lys spaced at n , n +1 and n +4 positions ( Supplementary Fig. S4 ). Such charged triplets are located one helical turn from each other, thus forming two salt bridges that are regarded as cooperative in nature, providing a more stabilizing effect than single salt bridges [29] . Additionally, there are also repulsive electrostatic interactions in the Beclin 1 CC domain structure that involve the three 'imperfect' charged residues at a position. These residues are adjacent to residues of the same electrostatic charge at the f position on the opposing peptide chain, forming a repulsive interaction across the dimer interface (E189 a- E249 e'′ , R203 a- K235 e' , E224 a -D221 e' ) ( Supplementary Fig. S4 ). Most notably the E224 a -D221 e' repulsive pair is located near the centre of the internal two-fold symmetry, creating a strong destabilizing effect at the central heptad repeat of the dimer structure ( Fig. 1e ). Beclin 1 CC domain is a metastable dimer To confirm that the dimeric state of the CC domain seen in our crystal structure reflects its oligomeric status in vitro , we characterized the CC domain by sedimentation equilibrium analytical ultracentrifugation. The sedimentation profile shows a single species with molecular weight of ∼ 21 kDa that matches a homodimer and corroborates our crystal structure of a dimeric CC ( Fig. 2a ). The unexpected large number of imperfect a - d' pairings observed at the dimer interface promoted us to assess the thermal stability of the CC domain by circular dichroism (CD) measurement at different temperatures ( Fig. 2b ). The CD spectrum of the CC domain at 20 °C shows a pattern with a double-bottom at wavelengths 222 and 208 nm that is characteristic of the CC structural motif [30] . At higher temperatures of 40 and 60 °C, there is a gradual loss of the double-bottom feature at 222 and 208 nm that probably implies disruption of the CC structure. The thermal transition temperature (or 'melting temperature' T m) of Beclin 1 CC domain, estimated by CD spectra, is ∼ 40 o C, indicating that the dimeric state is metastable at physiological temperature. The self dissociation constant ( K d ) of the Beclin 1 CC domain homodimer is ∼ 89 μM as estimated from isothermal titration calorimetry (ITC) experiments ( Supplementary Fig. S5 ). 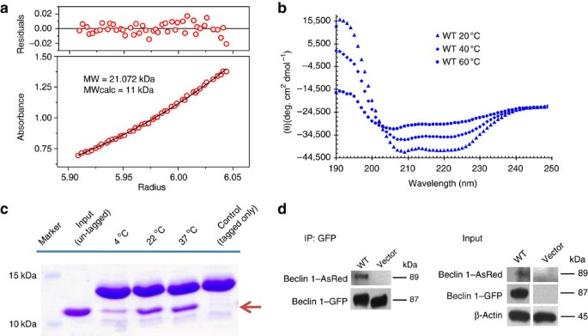Figure 2: The Beclin 1 CC domain is a metastable homodimer and mediates its self-associationin vivo.(a) The sedimentation equilibrium profile of the Beclin 1 CC domain. (b) The CD spectra of the Beclin 1 CC domain at different temperatures. (c). Dynamic exchange assay of wild-type Beclin 1. His-tagged and untagged Beclin 1 CC domain were co-incubated at the indicated temperatures and coprecipitated at preset temperatures by Ni2+– nitrilotriacetic acid (NTA) agarose beads. The presence of heterodimeric Beclin 1 CC domain, consisting of one monomer with his-tag and the other monomer without tag, was checked by SDS gel and indicated by the arrow. (d) Self-association pattern of Beclin 1in vivo. Both GFP- and AsRed-tagged full-length Beclin 1 are co-transfected into HEK 293T cells and their self-association is probed by co-IP using GFP antibody for immunoprecipitation, followed by western blot with anti-AsRed antibody. Figure 2: The Beclin 1 CC domain is a metastable homodimer and mediates its self-association in vivo. ( a ) The sedimentation equilibrium profile of the Beclin 1 CC domain. ( b ) The CD spectra of the Beclin 1 CC domain at different temperatures. ( c ). Dynamic exchange assay of wild-type Beclin 1. His-tagged and untagged Beclin 1 CC domain were co-incubated at the indicated temperatures and coprecipitated at preset temperatures by Ni 2+ – nitrilotriacetic acid (NTA) agarose beads. The presence of heterodimeric Beclin 1 CC domain, consisting of one monomer with his-tag and the other monomer without tag, was checked by SDS gel and indicated by the arrow. ( d ) Self-association pattern of Beclin 1 in vivo . Both GFP- and AsRed-tagged full-length Beclin 1 are co-transfected into HEK 293T cells and their self-association is probed by co-IP using GFP antibody for immunoprecipitation, followed by western blot with anti-AsRed antibody. Full size image To investigate whether the metastable Beclin 1 CC domain readily transits between dimer and monomer states, we carried out an exchange assay where two species of Beclin 1 CC domain, one with His 6 -tag and one without, were mixed together ( Fig. 2c ). The dynamic dissociation of metastable Beclin 1 CC domain and the exchange between the tagged and non-tagged homodimers should produce a heterodimeric species with one monomer carrying the His 6 -tag and the other monomer without. Indeed, for wild type, the presence of the heterodimeric Beclin 1 CC domain is noticeable even at 4 °C, and significantly increased at 22 and 37 °C, suggesting that the metastable Beclin 1 CC domain readily undergoes dynamic exchange between dimer and monomer states. To characterize the self association of Beclin 1 in vivo , GFP- and AsRed-tagged full-length Beclin 1 were co-transfected into HEK 293T cells and the interaction between the two tagged proteins was probed by co-immunoprecipitation (co-IP). GFP-tagged Beclin 1 could co-IP with AsRed-tagged Beclin 1, confirming the self-association of Beclin 1 in vivo ( Fig. 2d ). Furthermore, the bimolecular fluorescence complementation assay was used as an alternative method to directly visualize Beclin 1 self-association in vivo . Co-expression of Beclin 1-VN (Beclin 1 fused to the amino-terminal fragment of Venus, a YFP variant) and Beclin 1-VC (Beclin 1 fused to Venus C-terminal fragment) resulted in restoration of functional Venus and enhanced fluorescent signal, whereas co-expression of Beclin 1-VN and Beclin 1(ΔCE)-VC mutant with the CC domain deleted led to significantly reduced fluorescence in cells ( Supplementary Fig. S6 ). This result provides in vivo evidence for Beclin 1 self-interaction. Biophysically distinct Beclin 1–Atg14L/UVRAG heterodimers Both Atg14L and UVRAG contain CC regions that are essential for interaction with Beclin 1, possibly by forming an oligomeric CC assembly [18] , [19] , [21] . We proceeded to investigate how the metastable Beclin 1 CC domain interacts with the CC regions of Atg14L and UVRAG. The CC domain of Beclin 1 binds to the CC region of Atg14L and UVRAG in a highly exothermic fashion ( K d ∼ 3.22 and 0.24 μM, respectively), with stoichiometry of 1:1 as estimated from ITC measurements ( Fig. 3a,b ). The stoichiometry of the Beclin 1–Atg14L and Beclin 1–UVRAG complex was further analysed by sedimentation velocity analytical ultracentrifugation (Table 1). The Beclin 1 CC domain, as well as the CC region of Atg14L and UVRAG, were individually purified and mixed at different molar ratios ( Supplementary Fig. S7 ). The Atg14L CC region is monomeric, with the presence of a single peak of ∼ 11.1 kDa. A 1:1 Beclin 1:Atg14L mixture showed the presence of a single complex of ∼ 22.3 kDa, matching the sum of Beclin 1 monomer ( ∼ 11 kDa) and Atg14L CC region ( ∼ 11.5 kDa). A 1:5 Beclin 1:Atg14L mixture showed the presence of a peak of ∼ 11.6 kDa corresponding to the excessive Atg14L, which ensured that the other peak of ∼ 22.3 kDa corresponds to the Beclin 1–Atg14L heterodimer, not the Beclin 1 CC domain homodimer that has a similar molecular weight of ∼ 22 kDa. The sedimentation profile of 1:2 Beclin 1:UVRAG mixture also confirms a heterodimer with estimated molecular weight of ∼ 18.5 kDa, the sum of monomeric Beclin 1 ( ∼ 11 kDa) and UVRAG CC region ( ∼ 8.5 kDa). An excessive amount of UVRAG CC region was not directly detected, because it contains no aromatic residues for ultraviolet absorbance at 280 nm. Therefore, the metastable homodimeric form of Beclin 1 CC domain readily transits to stable heterodimeric Beclin 1–Atg14L/UVRAG complexes. 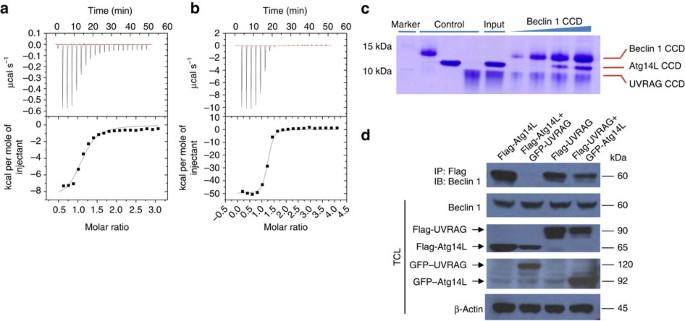Figure 3: The Beclin 1 CC domain forms heterodimeric complex with Atg14L and UVRAG with distinct biophysical properties. (a,b) ITC titration profile of Beclin 1 CC domain with Atg14L (a) or UVRAG (b). (c) Pull-down assay to assess the competition between Beclin 1–Atg14L and Beclin 1–UVRAG complexes. Increasing amount of His6-tagged Beclin 1 CC domain was added to a mixture of Atg14L and UVRAG proteins corresponding to their respective CC region. The Beclin 1–Atg14L/UVRAG complexes were pulled down by Ni2+– nitrilotriacetic acid (NTA) agarose beads and checked by SDS gel. (d) Co-IP experiments to assess the competition between Beclin 1–Atg14L and Beclin 1–UVRAG complexesin vivo. FLAG- or GFP-tagged Atg14L or UVRAG was transfected alone, or both were co-transfected into HEK 293T cells and their interaction with endogenous Beclin 1 was probed by co-IP using GFP antibody, followed by western blot with anti-Beclin 1 antibody. Figure 3: The Beclin 1 CC domain forms heterodimeric complex with Atg14L and UVRAG with distinct biophysical properties. ( a , b ) ITC titration profile of Beclin 1 CC domain with Atg14L ( a ) or UVRAG ( b ). ( c ) Pull-down assay to assess the competition between Beclin 1–Atg14L and Beclin 1–UVRAG complexes. Increasing amount of His 6 -tagged Beclin 1 CC domain was added to a mixture of Atg14L and UVRAG proteins corresponding to their respective CC region. The Beclin 1–Atg14L/UVRAG complexes were pulled down by Ni 2+ – nitrilotriacetic acid (NTA) agarose beads and checked by SDS gel. ( d ) Co-IP experiments to assess the competition between Beclin 1–Atg14L and Beclin 1–UVRAG complexes in vivo . FLAG- or GFP-tagged Atg14L or UVRAG was transfected alone, or both were co-transfected into HEK 293T cells and their interaction with endogenous Beclin 1 was probed by co-IP using GFP antibody, followed by western blot with anti-Beclin 1 antibody. Full size image Considering that Atg14L and UVRAG are two mutually exclusive binding partners of Beclin 1, and their association with Beclin 1 leads to formation of distinct Beclin 1–VPS34 complexes [17] , we proceeded to compare the biophysical properties of Beclin 1–Atg14L and Beclin–UVRAG interactions. UVRAG binds to Beclin 1 with stronger affinity than that of Atg14L ( K d 0.24 versus 3.22 μM). At high salt concentration of 1 M NaCl, the Beclin 1–UVRAG interaction, although weakened, is still detectable by ITC profile whereas the Beclin 1–Atg14L interaction is nearly lost ( Supplementary Fig. S8 ). These data suggest that the Beclin 1–UVRAG interaction is more hydrophobic in nature than the Beclin 1–Atg14L interaction. In the competitive binding assay by ITC experiments, UVRAG can successfully bind to Beclin 1 CC domain in the presence of Atg14L; whereas Atg14L fails to interact with CC domain in the presence of UVRAG ( Supplementary Fig. S9 ), suggesting that the Beclin 1–UVRAG interaction is of stronger affinity than that of Beclin 1–Atg14L interaction. The biophysical differences between Beclin 1–Atg14L and Beclin 1–UVRAG complexes were further characterized by in vitro and in vivo competition assays. When under-saturating amount of the Beclin 1 CC domain was added to a mixture of Atg14L and UVRAG CC proteins, the Beclin 1–UVRAG complex was preferentially formed ( Fig. 3c ). The Beclin 1–Atg14L complex was later detected, after an increasing amount of Beclin 1 was added to saturate UVRAG in the mixture. Furthermore, by co-transfecting Atg14L and UVRAG into HEK 293T cells and probing their interaction with endogenous Beclin 1 by co-IP, we found that overexpression of Atg14L had little impact on the formation of Beclin 1–UVRAG complex. In contrast, overexpression of UVRAG greatly reduced the amount of Beclin 1–Atg14L complex pulled down by co-IP ( Fig. 3d ). These data further demonstrate that the mutually exclusive Beclin 1–Atg14L and Beclin 1–UVRAG complexes have distinct biophysical properties, and that the Beclin 1–UVRAG interaction is noticeably stronger than that of Beclin 1–Atg14L. In summary, although the Beclin 1 CC domain is critical for mediating the formation of Beclin 1 homodimer, Beclin 1–Atg14L and Beclin 1–UVRAG heterodimer complexes, these three assemblies have distinct biophysical properties. The Beclin 1 homodimer is marked by its metastability and ready transition to the more stable heterodimeric Beclin 1–Atg14L/UVRAG complex with 1:1 stoichiometry. The Beclin 1–Atg14L and Beclin 1–UVRAG complexes compete for overlapping interaction sites in the Beclin 1 CC domain, yet UVRAG readily outcompetes Atg14L for association with Beclin 1 owing to its stronger affinity. CC mutants in monomeric and stabilized dimer forms To test the functional importance of the metastability of the CC domain in mediating Beclin 1–Atg14L/UVRAG interaction, we generated two classes of mutants, the monomeric class (MutM) that are designed to adopt a monomeric form after the canonical hydrophobic a - d' pairings, critical for dimer formation, are weakened; and the stabilized class (MutStab) that are designed to be a 'stabilized' dimer with imperfect a - d' pairings modified to enhance homodimer stability and impair its transition into Beclin 1–Atg14L/UVRAG heterodimer. For MutM constructs, we generated double mutants of L178A/L259A, L178A/L192A and L178A/L196A to weaken the three 'leucine zippers' at the dimer interface ( Fig. 4a ). For MutStab constructs, we mutated the three charged residues found in the 'imperfect' a - d' pairings (E189, E224 and R203) that are perceived to cause the most destabilizing effect to canonical hydrophobic Leu residues to stabilize the dimeric state, whereas the combination of these mutations of charged residues with further mutations of A217L and A255L to generate double (E189L/A255L and A217L/E224L), triple (A217L/E224L/A255L) or quadruple mutants (E189L/A217L/E224L/A255L) would further enhance the dimer stability ( Fig. 4a ). 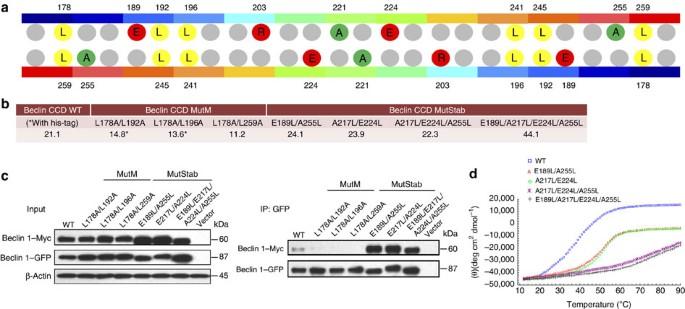Figure 4: Characterization of Monomeric (MutM) and Stabilized (MutStab) Mutants of Beclin 1 CC Domain. (a) The scheme for designing monomeric (MutM) or stabilized (MutStab) mutants of the Beclin 1 CC domain. Wild-type CC domain dimer is represented in the centre as two antiparallel colour bars. Each individually coloured segment on the two bars represents a single heptad repeat. The colour gradient is from blue at N-terminal to red at C-terminal. Two grey spheres are drawn for each coloured segment, indicating theaanddresidues that form the dimer interface. The canonicala-d'pairings mutated in MutM constructs are coloured yellow and the imperfecta-d'pairings mutated in MutStab constructs are coloured red for charged residues or green for alanine residues. (b) The estimated molecular weight of Beclin 1 CC domain wild-type, MutM and MutStab constructs based on their respective sedimentation equilibrium profile (Supplementary Fig. S10). (c) Self-association pattern of wild-type, MutM and MutStab constructs of Beclin 1in vivo. For each construct, both GFP- and Myc-tagged full-length Beclin 1 are co-transfected into HEK 293T cells and their self-association is probed by co-IP using GFP antibody for IP, followed by western blot with anti-Myc antibody. (d). Temperature-dependent CD profile of Beclin 1 CC domain wild-type and MutStab constructs at 220 nm. Figure 4: Characterization of Monomeric (MutM) and Stabilized (MutStab) Mutants of Beclin 1 CC Domain. ( a ) The scheme for designing monomeric (MutM) or stabilized (MutStab) mutants of the Beclin 1 CC domain. Wild-type CC domain dimer is represented in the centre as two antiparallel colour bars. Each individually coloured segment on the two bars represents a single heptad repeat. The colour gradient is from blue at N-terminal to red at C-terminal. Two grey spheres are drawn for each coloured segment, indicating the a and d residues that form the dimer interface. The canonical a - d' pairings mutated in MutM constructs are coloured yellow and the imperfect a - d' pairings mutated in MutStab constructs are coloured red for charged residues or green for alanine residues. ( b ) The estimated molecular weight of Beclin 1 CC domain wild-type, MutM and MutStab constructs based on their respective sedimentation equilibrium profile ( Supplementary Fig. S10 ). ( c ) Self-association pattern of wild-type, MutM and MutStab constructs of Beclin 1 in vivo . For each construct, both GFP- and Myc-tagged full-length Beclin 1 are co-transfected into HEK 293T cells and their self-association is probed by co-IP using GFP antibody for IP, followed by western blot with anti-Myc antibody. ( d ). Temperature-dependent CD profile of Beclin 1 CC domain wild-type and MutStab constructs at 220 nm. Full size image The oligomeric state of each MutM or MutStab mutant was analysed via sedimentation equilibrium analytical centrifugation ( Fig. 4b , Supplementary Fig. S10 ). Indeed, all CC domain mutants of MutM class behave as monomeric species with estimated molecular weight of ∼ 11 kDa. The single-, double- and triple-mutant MutStab behave as dimeric species with molecular weight of ∼ 22 kDa whereas the quadruple MutStab construct (E189L/A217L/E224L/A255L) seems to oligomerize further in tetrameric form, which might be owing to nonspecific higher order self-association. To confirm the self-association pattern of the various Beclin 1 mutants in vivo , we expressed their full-length mutant constructs in HEK 293T cells. For each mutant, a GFP-tagged version was co-transfected with a Myc-tagged version, followed by co-IP. As expected, a GFP-MutM mutant cannot co-IP with Myc-MutM carrying the same mutation, confirming that the MutM mutants are monomeric in vivo ( Fig. 4c ). In contrast, the GFP-tagged wild-type and MutStab mutants readily co-IP with their respective Myc-tagged partner, suggesting that wild-type and MutStab mutants self associate in vivo . To assess whether the MutStab have enhanced thermal stability, the CD spectra of wild type and MutStab were measured at different temperatures ( Fig. 4d ). The thermal transition temperature for MutStab CC domain were significantly enhanced over that of wild-type Beclin 1, as indicated with T m for double mutants at ∼ 45 °C and for triple and quadruple mutants at higher than 60 °C. This data confirm that the MutStabs have significantly enhanced thermal stability over the metastable wild type after more than one of their imperfect a - d' pairs have been replaced by canonical residues. To investigate whether the MutStab have impaired homodimer–heterodimer transition, the exchange assay was performed as previously described ( Supplementary Fig. S11 ). For MutStab, the E189L/A255L mutant has reduced, but still noticeable, exchange in a temperature-dependent manner, whereas the A217L/E224L, the triple, and the quadruple mutants have completely lost their exchange. Taken together, our MutM constructs with perfect a - d' pairings at the dimer interface of CC domain weakened produce monomeric Beclin 1, whereas the MutStab constructs with imperfect a - d' pairings improved produce dimeric Beclin 1 with enhanced thermostability. Monomeric mutants retain interaction with Atg14L and UVRAG We next characterized the interaction of MutM and MutStab with Atg14L and UVRAG. The interactions of MutM CC domains with Atg14L and UVRAG were first assessed by ITC assays. The three CC MutM constructs L178A/L259A, L178A/L192A and L178A/L196A all show very similar K d and stoichiometry values to that of wild type, suggesting that this group of mutants interact strongly with Atg14L and UVRAG in similar fashion to wild type ( Table 1 ). Table 1 Summary of the binding affinity ( K d) and stoichiometry of for Beclin1-Atg14L/UVRAG interaction as measured by ITC and analytic ultracentrifugation experiments. Full size table We further investigated the interaction of Beclin 1 MutM mutants with Atg14L and UVRAG in cultured cells. We expressed GFP–Beclin 1 variants (including wild-type and MutM mutations) alone or together with FLAG-UVRAG in HEK 293T cells and assessed by co-IP assay the interaction of Beclin 1 with endogenous Atg14L ( Fig. 5a ) or FLAG-UVRAG ( Fig. 5b ), respectively. The wild-type GFP–Beclin 1 and MutMs L178A/L192A, L178A/L196A and L178A/L259A co-IP in a similar efficiency with endogenous Atg14L or FLAG-UVRAG. Taken together, the result demonstrates that the Beclin 1 mutants defective in homodimer formation are not affected in Beclin 1–Atg14L or Beclin 1–UVRAG heterodimer formation. Therefore, the monomeric form of Beclin 1 is sufficient for interaction with Atg14L and UVRAG. 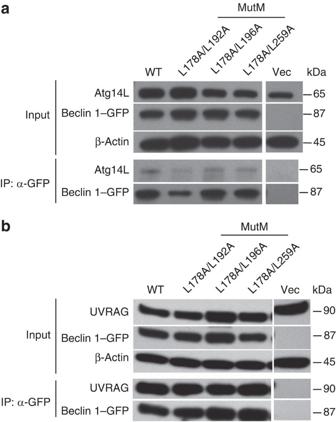Figure 5: Monomeric (MutM) mutants of Beclin 1 CC domain retain interaction with Atg14L and UVRAG. (a,b) Interaction of Beclin 1 wild-type and monomeric (MutM) mutants with Atg14L or UVRAG in cultured cells. HEK 293T cells were transfected with GFP-tagged Beclin 1 variant alone (a) or together with FLAG-UVRAG (b). The lysates were immunoprecipitated by GFP antibody, followed by western-blot analysis with anti-Atg14L antibody for detecting binding to endogenous Atg14L (a) or with anti-UVRAG antibody for detecting binding to the FLAG-tagged UVRAG protein (b). Figure 5: Monomeric (MutM) mutants of Beclin 1 CC domain retain interaction with Atg14L and UVRAG. ( a , b ) Interaction of Beclin 1 wild-type and monomeric (MutM) mutants with Atg14L or UVRAG in cultured cells. HEK 293T cells were transfected with GFP-tagged Beclin 1 variant alone ( a ) or together with FLAG-UVRAG ( b ). The lysates were immunoprecipitated by GFP antibody, followed by western-blot analysis with anti-Atg14L antibody for detecting binding to endogenous Atg14L ( a ) or with anti-UVRAG antibody for detecting binding to the FLAG-tagged UVRAG protein ( b ). Full size image Specific binding of stabilized mutants to Atg14L versus UVRAG By using ITC assays and co-IP experiments, we found that the MutStab Beclin 1 mutants have distinct interaction profiles with Atg14L versus UVRAG. ITC results showed that nearly all MutStab mutants of Beclin 1 CC domains have lost their interaction with Atg14L ( Table 1 and Supplementary Fig. S12 ). Only the single-mutant MutStab E224L shows residual interaction with Atg14L as judged by the significantly weakened exothermic profile in ITC measurement ( Supplementary Fig. S12 ). In contrast, nearly all MutStab CC domains clearly retain, albeit reduced, interaction with UVRAG as compared with wild type. The K d values of the double mutants are approximately weakened by 5–10 times, whereas the stoichiometry is ∼ 1:1 as estimated from ITC experiments. The triple- and quadruple-mutants show further weakened interaction with UVRAG as compared with the single- and double-mutants. Only the single-mutant MutStab R203L has no detectable exothermic interaction with UVRAG as judged by the ITC profile ( Supplementary Fig. S12 ). We also examined the interaction of full-length Beclin 1 MutStab mutants with Atg14L and UVRAG in cultured cells. We co-expressed GFP–Beclin 1 variants (including wild-type, double-mutant E189L/A255L and quadruple mutant E189L/A217L/E224L/A255L) alone or together with FLAG-UVRAG in HEK 293T cells and assessed by co-IP assay, the interaction of Beclin 1 with endogenous Atg14L ( Fig. 6a ) and FLAG-UVRAG ( Fig. 6b ) respectively. The interaction of Atg14L with Beclin 1 MutStab E189L/A255L is reduced; whereas the interaction with MutStab E189L/A217L/E224L/A255L is significantly impaired. By contrast, FLAG-UVRAG co-IP with the two GFP–Beclin 1 MutStab mutants with a similar efficiency to GFP–Beclin 1 wild type. As noted, although mutants E189L/A255L and E189L/A217L/E224L/A255L had no binding to Atg14L CC region or reduced interaction with UVRAG CC region in ITC assay, the full-length Beclin 1 carrying the same mutations did not completely lose the interaction with Atg14L or did not change significantly the binding to UVRAG based on the co-IP analysis. This result may reflect the different assay conditions in the two studies or the sequence region outside Beclin 1-CCD, Atg14L-CCD or UVRAG-CCD that may also influence the interactions. 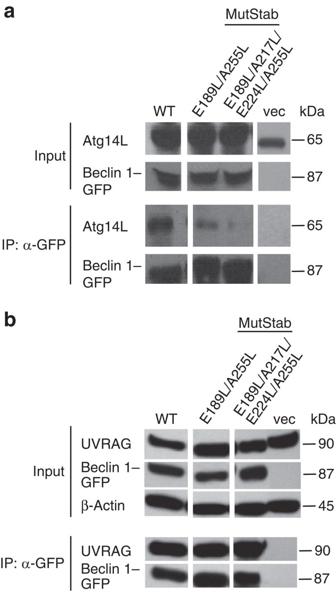Figure 6: Difference in the binding of stabilized (MutStab) mutants of Beclin 1 CC to Atg14L or UVRAG. (a,b) Interaction of MutStab mutants of Beclin 1 with Atg14L or UVRAGin vivo. HEK 293T cells were transfected with GFP-tagged Beclin 1 variant alone (b) or together with FLAG-UVRAG (b). The lysates were immunoprecipitated by GFP antibody, followed by western blot analysis with anti-Atg14L antibody for detecting binding to endogenous Atg14L (a) or with anti-UVRAG antibody for detecting binding to the FLAG-tagged UVRAG protein (b). Figure 6: Difference in the binding of stabilized (MutStab) mutants of Beclin 1 CC to Atg14L or UVRAG. ( a , b ) Interaction of MutStab mutants of Beclin 1 with Atg14L or UVRAG in vivo . HEK 293T cells were transfected with GFP-tagged Beclin 1 variant alone ( b ) or together with FLAG-UVRAG ( b ). The lysates were immunoprecipitated by GFP antibody, followed by western blot analysis with anti-Atg14L antibody for detecting binding to endogenous Atg14L ( a ) or with anti-UVRAG antibody for detecting binding to the FLAG-tagged UVRAG protein ( b ). Full size image Subcellular localization of Beclin 1 mutants and Atg14L/UVRAG In a previous study, we showed that simultaneous overexpression of Beclin 1 and Atg14L in transfected cells promoted the co-localized Beclin 1–Atg14L puncta and recruited early autophagosomes marker [19] . Using this assay, we examined the localization of co-expressed AsRed–Atg14L and Beclin 1–GFP variants. As expected, AsRed–Atg14L and wild-type Beclin 1–GFP co-localized in intracellular discrete puncta. Similar to wild-type Beclin 1, the GFP–Beclin 1 MutM L178A/L192A also formed puncta with AsRed–Atg14L. By contrast, GFP–Beclin 1 MutStabs, E189L/A255L and E189L/A217L/E224L/A255L, are largely diffused when co-expressed with AsRed–Atg14L ( Fig. 7a ). This result indicates that Beclin 1 MutMs retain the ability to bind Atg14L and promote autophagosome formation, whereas Beclin 1 MutStabs are defective in interaction with Atg14L, and perhaps impaired in autophagy regulation. However, co-expression of UVRAG and Beclin 1 variants (including Beclin1 wild type, all MutM and MutStab mutants) led to diffused fluorescent signalling throughout cytoplasm ( Fig. 7b ). Taken together, the results suggest that the Beclin 1–Atg14L interaction is highly sensitive to the metastable imperfect dimer interface of Beclin 1. The monomeric form (MutMs) with the imperfect residues at the dimer interface retained co-localize with Atg14L. In contrast the stabilized dimeric form (MutStabs) with the imperfect residues altered can not. In contrast, the Beclin 1–UVRAG interaction is less sensitive to the imperfect dimer interface of Beclin 1 and seems to have a cellular localization profile distinct from that of the Beclin 1–Atg14L interaction. 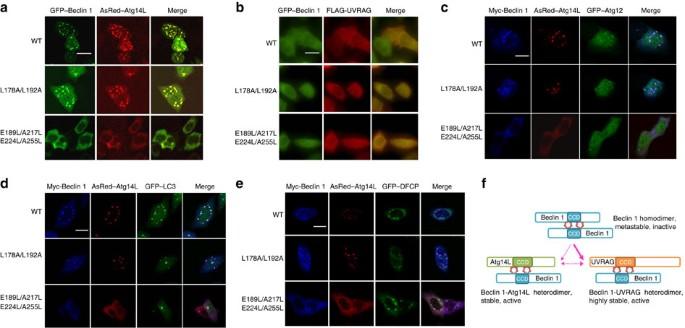Figure 7: Subcellular localization of Beclin 1 MutM and MutStab with co-expressed Atg14L or UVRAG proteins and early autophagosome markers. (a,b). Representative fluorescent images of HeLa cells co-tansfected with GFP-tagged Beclin 1 wild type, MutM L178A/L192A or MutStab E189L/A217L/E224L/A255L (green) and AsRed–Atg14L (red) (a) or FLAG-UVRAG (red) (b); Co-localization of AsRed–Atg14L with GFP-tagged Beclin 1 wild type or MutM is shown in discrete puncta. (c–e) Representative fluorescence images of HeLa cells co-transfected with Myc-Beclin 1 wild type, MutM L178A/L192A or MutStab E189L/A217L/E224L/A255L (blue), AsRed–Atg14L (red) and GFP-tagged Atg12 (c), LC3 (d) and DFCP (e) (green). The scale bar is 20 μM. (f). A proposed model for the dynamic transition among homodimer (antiparallel) of Beclin 1, and the heterodimers of Beclin 1–Atg14L and Beclin 1–UVRAG. Multiple homo- and hetero-oligomeric forms of Beclin 1 protein exist intracellularly, and the nature of metastability in Beclin 1 CCD interface facilitates the transition of Beclin 1 homodimer to Beclin 1–Atg14L/UVRAG heterodimer that are compatible with activated autophagy-lysosomal degradation. The star shapes indicate the imperfect dimer interface. The thicker arrows pointing towards Beclin 1–UVRAG complex indicate its stronger affinity. Figure 7: Subcellular localization of Beclin 1 MutM and MutStab with co-expressed Atg14L or UVRAG proteins and early autophagosome markers. ( a , b ). Representative fluorescent images of HeLa cells co-tansfected with GFP-tagged Beclin 1 wild type, MutM L178A/L192A or MutStab E189L/A217L/E224L/A255L (green) and AsRed–Atg14L (red) ( a ) or FLAG-UVRAG (red) ( b ); Co-localization of AsRed–Atg14L with GFP-tagged Beclin 1 wild type or MutM is shown in discrete puncta. ( c–e ) Representative fluorescence images of HeLa cells co-transfected with Myc-Beclin 1 wild type, MutM L178A/L192A or MutStab E189L/A217L/E224L/A255L (blue), AsRed–Atg14L (red) and GFP-tagged Atg12 ( c ), LC3 ( d ) and DFCP ( e ) (green). The scale bar is 20 μM. ( f ). A proposed model for the dynamic transition among homodimer (antiparallel) of Beclin 1, and the heterodimers of Beclin 1–Atg14L and Beclin 1–UVRAG. Multiple homo- and hetero-oligomeric forms of Beclin 1 protein exist intracellularly, and the nature of metastability in Beclin 1 CCD interface facilitates the transition of Beclin 1 homodimer to Beclin 1–Atg14L/UVRAG heterodimer that are compatible with activated autophagy-lysosomal degradation. The star shapes indicate the imperfect dimer interface. The thicker arrows pointing towards Beclin 1–UVRAG complex indicate its stronger affinity. Full size image We further analysed the co-localization of Beclin 1 and Atg14L with autophagosome-related markers. We found that co-expression of AsRed–Atg14L and GFP–Beclin 1 wild-type or MutM L178A/L192A caused the recruitment of GFP–DFCP (omegasome marker), GFP–Atg12 (early autophagosome marker) and GFP–LC3 (autophagosome marker) signals to proximity of Beclin 1/Atg14L puncta, whereas MutStab are diffuse in cytoplasm and do not show co-localization with those GFP reporters ( Fig. 7c-e ). The data provide further support to our conclusion that Beclin 1 MutMs are similar to wild type in the ability to form a complex with Atg14L and to promote autophagosome synthesis. In contrast, the MutStabs are impaired in Atg14L binding and autophagosome synthesis. Previous studies and our experiments demonstrate that Beclin 1 forms a dimer in vitro and in vivo as mediated by its CC domain [18] , [19] , [20] , [31] , [32] . Here we show that the crystal structure of Beclin 1 CC domain is an antiparallel dimeric CC with the unexpected characteristic of containing a series of 'imperfect' a - d' pairings at its dimer interface. These 'imperfect' pairs render the dimeric state of Beclin 1 metastable and facilitate its transition to form heterodimeric Beclin 1–Atg14L/UVRAG complexes. Strengthening Beclin 1 dimer stability by modifying the imperfect a - d' pairs leads to significant loss or reduction of interaction with Atg14L and UVRAG and impaired autophagosome synthesis, whereas reducing Beclin 1 dimer stability and locking it in monomeric form by disrupting canonical hydrophobic a - d' pairs does not affect its interaction with Atg14L or UVRAG. Our findings suggest a dynamic exchange among three Beclin 1 complexes, that is, its homodimer and the Atg14L- or UVRAG-containing heterodimeric complexes driven by their distinct biophysical affinities ( Fig. 7f ). Beclin 1 homodimer, with the weakest association strength among these three, readily transits into Atg14L- or UVRAG-containing complexes in the presence of either binding partner. UVRAG, with its stronger affinity for Beclin 1 as compared with that of Atg14L, may drive the formation of Beclin 1–UVRAG complex at the expense of Atg14L. Thus, the balance among these multiple complexes can be influenced by the relative abundance of Beclin 1, Atg14L and UVRAG. We propose that a fraction of intracellular Beclin 1 exists in homodimer [31] , [32] , particularly considering that both Atg14L- and UVRAG-containing Beclin 1–VPS34 complexes have been detected even though the Beclin 1–UVRAG complex has stronger affinity; however, the biological significance of the homodimeric Beclin 1 is unclear. It is tempting to propose that homodimeric Beclin 1, perhaps as a reserve pool, remain inactive; on autophagy induction or related signals, Beclin 1 can be triggered to undergo transition from inactive homodimer to heterodimeric Beclin 1–Atg14L/UVRAG formation that may be correlated with enhanced lipid kinase activity of VPS34 to promote autophagy. We further postulate that the existence of such a homodimer pool of Beclin 1 and its flexibility in homodimer–heterodimer transition to form distinct Beclin 1–VPS34 subcomplexes is an important part of regulatory mechanism for Beclin 1 in promoting a highly efficient autophagy activation/lysosomal degradation at levels of protein complex decomposition/reassembly without invoking gene transcription and protein synthesis. This flexibility in transition and the dynamic re-distribution of Beclin 1 among its self-associated form or Atg14L/UVRAG-containing Beclin 1–VPS34 subcomplexes relies critically on the metastability of Beclin 1, as determined by the imperfect dimer interface of its CC domain. A previous study by Noble et al . reported similar dimer–monomer transition for Beclin 1 induced by UVRAG [32] . Their data also suggest that the anti-apoptotic Bcl2 family of proteins may inhibit autophagy by stabilizing Beclin 1 homodimer conformation, thus impeding its interaction with autophagy-activating factor such as UVRAG. Further studies are required to confirm such regulation mechanism; particularly, how such regulation is implemented by the various Beclin 1-interacting regulatory factors of VPS34 activity such as Bif-1, Rubicon, Ambra1 and so on. In this study, we also noticed the distinct role for the imperfect and metastable dimer interface of Beclin 1 in mediating its interaction with Atg14L and UVRAG, respectively. The charged residues of the imperfect a - d' pairings (E189, R203 and E224) are directly involved in Beclin 1–Atg14L interaction because mutating these amino acids to hydrophobic leucine residue nearly abolishes or reduces Beclin 1–Atg14L interaction. Yet, MutStab E189L and E224L retain interaction with UVRAG similar to the wild-type Beclin 1. Combining E189L and E224L mutations with extra mutations (A217L and A255L) leads to further reduction of interaction with UVRAG and noticeably enhanced dimer stability. Thus, the charged residues E189 and E224 likely indirectly mediate Beclin 1–UVRAG interaction by affecting the Beclin 1 dimer stability and its transition to heterodimeric Beclin 1–UVRAG complex. Although the detailed mechanism of Beclin 1–Atg14L/UVRAG interaction remains to be further shown, our study starts to provide insight into the structural basis for how Beclin 1 differentially interacts with multiple binding partners. This information will be central to the understanding of molecular mechanism that controls the formation of various Beclin 1–VPS34 subcomplexes to exert their effect on arrays of VPS34-related activities including autophagy. Protein expression and purification The CC domain of rat Beclin 1 (residues 174–266) was cloned as a His 6 -tagged protein in a modified pET32 vector containing the human rhinovirus 3C protease cleavage site and without thioredoxin fusion. The MutM (L178A/L259A, L178/L192A and L178A/L196A) and MutStab constructs (E189L/A255L, A217L/E224L, A217L/E224L/A255L and E189L/A217L/E224L/A255L) of the CC domain were generated by site-directed mutagenesis (Finnzyme) and cloned into the same vector as wild type. Wild-type and mutant CC domain constructs were expressed in Escherichia coli BL21 (DE3) cells at 30 °C after induction by isopropyl-β-d-thiogalactopyranoside and purified by affinity chromatography (HisTrap HP, GE Healthcare). The His 6 tag was removed by 3C cleavage and the untagged protein was further purified by size-exclusion chromatography (Superdex 75, GE Healthcare). For dimer exchange assay, the His 6 -tagged version of Beclin 1 CC domain was produced by cloning it into pRSETA vector (Invitrogen) that does not contain 3C cleavage site. Both wild-type and MutStab constructs (E189L/A255L, A217L/E224L, A217L/E224L/A255L and E189L/A217L/E224L/A255L) were cloned into this vector. The His 6 -tagged CC domain constructs were expressed under the same condition as un-tagged version, and purified by affinity column chromatography with no protease cleavage. The CC region of rat Atg14L (residues 88–178) was cloned as GST-fusion His 6 -tagged protein into a modified pET32 vector (Novagen) containing the 3C protease cleavage site. The CC region of mouse UVRAG (residues 228–298) was cloned as thioredoxin-fusion His 6 -tagged protein to the same modified pET-49b(+) vector (Novagen) as used for Beclin 1 CC domain. Both constructs were expressed at 30 °C in E . coli BL21 (DE3) cells after isopropyl-β-d-thiogalactopyranoside induction and purified by affinity chromatography (HisTrap HP, GE Healthcare). Further purification after 3C cleavage was carried out using size-exclusion chromatography (Superdex 75, GE Healthcare). Crystallization and structure determination Crystals were grown at 16 °C by the hanging drop vapour diffusion method mixing 1 μl of Beclin 1 CC domain at 50 ∼ 52 mg ml −1 with 1 μl of reservoir solution containing 45% 2-methyl-2,4-pentadiol, 2% PEG400, and 100 mM Tris buffer (pH 8.2). The Au derivative was obtained by soaking crystals in reservoir solution containing 2 mM AuCl 4 for 2 h. The iodine derivative was obtained by growing crystals in reservoir solution with 300 mM NH 4 I added. All data were collected at 100 K on our in-house X-ray system (MicroMax 007 HF, Rigaku), indexed and integrated by MOSFLM [33] , and scaled by the SCALA module [34] in the CCP4 suite ( http://www.ccp4.ac.uk/ ) [35] . The Au and iodine sites were located and refined using SOLVE [36] and further refined using MLPHARE and DM [37] modules in CCP4 to build an interpretable electron density map. The structure was built manually using COOT [38] and the final structure was refined using REFMAC [39] module in CCP4. Statistics were summarized in Supplementary Table S1 . The coordinates of Beclin 1 CC domain has been deposited to Protein Data Bank (PDB ID 3Q8T). The structure figures were prepared using the CCP4 mg package [40] in CCP4. Analytical ultracentrifugation Sedimentation velocity experiments were performed using a ProteomeLab XL-A analytical ultracentrifuge (Beckman Coulter) with two-channel centre-pieces in an An-60Ti rotor at 142,000 g and at 25 °C. Radial scans were measured at 280 nm. The solvent density and viscosity as well as the protein partial specific volume were calculated using the program SEDNTERP. The data were fitted to the continuous size-distribution functions c(S) using the program SEDFIT. Sedimentation equilibrium experiments were performed using a ProteomeLab XL-A analytical ultracentrifuge using six-channel centrepieces in an An-60Ti rotor at 25 °C. Three protein samples with different concentration were centrifuged until they reached equilibrium and no further change was seen in the distribution. Radial scans were measured at 280 nm. The final sedimentation equilibrium data were analysed using the XL-A/XL-I data analysis software provided by the manufacturer. Circular dichroism spectroscopy CD full-length scanning spectra were collected between 190 and 250 nm at 20 °C using a quartz cell with a 0.1 cm path length on a Jasco J-810 spectropolarimeter equipped with thermoelectric temperature control. Measurements were made on protein samples at 50 μM concentration in 50 mM NaCl, 20 mM Tris buffer, pH 8.0. Spectra were collected at 1.0 nm intervals with a 5-s averaging time per data point. A reference spectrum generated from a scan of the buffer without sample was subtracted before data were converted to mean residue ellipticity. Melting temperature spectra were collected between 12 and 90 °C at 222 nm. The temperature increment was 1 °C, the equilibration time 3 min and the average time 1 min. Dimer exchange assay For formation of heterodimer on exchange between differently tagged homodimer, His 6 -tagged and untagged Beclin CC domain was incubated together in ∼ 1:2 molar ration at varying temperatures for 20 min in 250 μl volume of binding buffer (150 mM NaCl, 50 mM Tris buffer, pH 8.0, 40 mM imidazole). Samples were flash-frozen in liquid N 2 to capture the resulting association state, and then thawed on ice. Ni 2+ -NTA agarose beads, pre-equilibrated with chilled binding buffer, were added to samples, which were then centrifuged to co-precipitate Ni 2+ -NTA beads with bound proteins. After thorough wash, the bound protein was eluted by SDS sample buffer and analysed by SDS–PAGE. Isothermal titration calorimetry Isothermal Titration Calorimetry was performed using an iTC200 microcalorimeter (MicroCal). Samples were dialysed into 50 mM Tris, pH 8.0, and 150 mM NaCl (or 1 M NaCl for high-salt condition). For Beclin 1–Atg14L/UVRAG interactions, the injection syringe was loaded with 40 μl of Beclin 1 sample and the cell was loaded with 220 μl of Atg14L/UVRAG sample. For the competitive assay, the preformed saturated complex of Beclin 1–Atg14L/UVRAG (with Atg14L/UVRAG being excessive) were loaded into the cell and the competing sample of UVRAG/Atg14L was loaded into the injection syringe. Typically, titrations consisted of 20 injections of 2 μl, with 180-s equilibration between injections. The data were analysed using Origin 7.0. In vitro competition assay Purified CC region of Atg14L and UVRAG at 20 μM concentration and 1:1 molar ratio were mixed in binding buffer (150 mM NaCl, 50 mM Tris buffer, pH 8.0). Purified His 6 -tagged Beclin 1 CC domain was added to the Atg14L-UVRAG mixture at increasing molar ratio of 0.1:1:1, 1:1:1, 4:1:1 and 20:1:1 and incubated at room temperature for 30 min. The Beclin 1–Atg14L-UVRAG mixture was then subject to standard procedure of pull-down experiment procedure using Ni 2+ -NTA agarose beads. After thorough wash, the bound protein was eluted by SDS sample buffer and analysed by SDS–PAGE. Immunoprecipitation DNA plasmids were transfected into HEK 293T cells. For co-IP experiments demonstrating self-association, GFP-tagged Beclin 1 plasmids were co-transfected with AsRed- or Myc-tagged Beclin 1 plasmids in equal amounts. For co-IP experiments demonstrating Beclin 1–Atg14L/UVRAG interaction, GFP-tagged Beclin 1 plasmids or equal amounts of GFP-tagged Beclin 1 plasmids and FLAG-UVRAG were transfected to test interaction with endogenous Atg14L or co-transfected UVRAG, respectively. For co-IP experiments demonstrating competition between Atg14L and UVRAG for interaction with endogenous Beclin 1, FLAG- and GFP-tagged Atg14L and UVRAG were transfected alone or co-transfected. Cells were lysed in IP lysis buffer (20 mM HEPES/pH7.4, 1 mM MgCl 2 , 0.25 mM CaCl 2 , 0.1% Triton X-100, 120 mM NaCl, EDTA-free protease inhibitor cocktail (Roche), 200 μg ml −1 phenylmethylsulfonyl fluoride, pepstatin 4 μg ml −1 , and DNase I). Lysates were incubated with GFP antibody overnight at 4 °C and then incubated with Dynabeads protein G (Invitrogen) for 1 h. The beads were washed in 1× IP lysis buffer 5 times and then eluted with 2× SDS sample buffer. Fluorescent microscopy imaging HeLa cells were maintained in DMEM supplemented with 10% fetal bovine serum and 1% penicillin–streptomycin (Invitrogen). Transient DNA transfection was performed using Lipofectamine 2000 (Invitrogen), following manufacturer's protocol. Cells were fixed in fresh 4% paraformaldehyde for 10 min, and permeablized with 0.1% Triton X-100 in PBS for 15 min at room temperature. After blocking in PBS containing 5% BSA for 30 min, cells were incubated in primary antibodies for 1 h. After three washes in PBS, cells were incubated with fluorescent secondary antibodies for one hour at room temperature, followed by four washes in PBS. Cells were mounted with fluorescence mounting medium and examined under confocal microscopes. The objective lens 63X was used for imaging. Acccession codes: The coordinates of Beclin 1 CC domain have been deposited in the Protein Data Bank under accession code PDB ID 3Q8T . How to cite this article: Li, X. et al . Imperfect interface of Beclin1 coiled-coil domain regulates homodimer and heterodimer formation with Atg14L and UVRAG. Nat. Commun. 3:662 doi: 10.1038/ncomms1648 (2012).